Scanning STED-FCS reveals spatiotemporal heterogeneity of lipid interaction in the plasma membrane of living cells The interaction of lipids and proteins plays an important role in plasma membrane bioactivity, and much can be learned from their diffusion characteristics. Here we present the combination of super-resolution STED microscopy with scanning fluorescence correlation spectroscopy (scanning STED-FCS, sSTED-FCS) to characterize the spatial and temporal heterogeneity of lipid interactions. sSTED-FCS reveals transient molecular interaction hotspots for a fluorescent sphingolipid analogue. The interaction sites are smaller than 80 nm in diameter and lipids are transiently trapped for several milliseconds in these areas. In comparison, newly developed fluorescent phospholipid and cholesterol analogues with improved phase-partitioning properties show more homogenous diffusion, independent of the preference for liquid-ordered or disordered membrane environments. Our results do not support the presence of nanodomains based on lipid-phase separation in the basal membrane of our cultured nonstimulated cells, and show that alternative interactions are responsible for the strong local trapping of our sphingolipid analogue. Resolving the various interactions of lipids and proteins in the eukaryotic plasma membrane (such as the possible formation of ‘lipid rafts’) with high temporal and spatial resolution is at the basis of understanding its diverse functions [1] . However, decoding the multitudes of interactions between membrane proteins and lipids in the living cell has been hampered by the lack of appropriate methods (for example, ref. 1 ). A prominent approach to reveal molecular interactions in the plasma membrane of living mammalian cells is studying diffusion of lipids and proteins. Here the challenge is to noninvasively observe the molecular mobility with (i) single-molecule sensitivity, (ii) a spatial resolution at the macromolecular scale and (iii) a temporal resolution on the submillisecond range. We have previously introduced the combination of subdiffraction resolution stimulated emission depletion (STED) microscopy [2] , [3] with single-molecule-based fluorescence correlation spectroscopy (FCS; STED-FCS) [4] , matching all of the above requirements. STED-FCS enabled the direct observation of millisecond anomalous lipid and protein dynamics on spatial scales down to ∼ 30 nm, that is about an order of magnitude below the diffraction resolution limit of far-field light microscopy [5] , [6] , [7] , [8] , [9] . Specifically, these experiments have shown hindered diffusion of various fluorescent lipid analogues when incorporated into the plasma membrane of live mammalian cells. Only STED but not standard confocal FCS measurements revealed that these hindrances were because of transient interactions with immobile or slowly moving molecular entities, presumably proteins. For the diffusing lipid analogues, this resulted in lipid-specific transient arrests or traps, which lasted between 1 and 10 ms [5] , [6] , [7] , [9] , [10] . While these transient arrests could involve several molecules, the area in which the lipids dwelled during trapping were smaller than 20 nm in diameter [5] , [6] , [7] , [9] , [10] . Yet, the impact of the observed lipid interactions on cellular functionality still remains to be investigated, especially their relation to lipid nanodomains or ‘lipid rafts’. The ‘lipid raft’ concept links the ability of lipids and proteins to segregate into liquid-ordered membrane phases with their need to form transient molecular complexes during cellular signalling [1] , [7] , [11] . Therefore, an important issue is to characterize the sites of lipid interactions. In particular, we need to understand how these involve liquid-disordered and -ordered membrane environments, and how they change over space and time. Unfortunately, mostly liquid-disordered preferring fluorescent lipid analogues have been investigated in high-resolution studies so far. In addition, an accurate spatiotemporal characterization of the lipid interactions was impossible by our previous STED-FCS measurements, since these only allowed the acquisition of data at one single small observation spot at a time. The simultaneous recording of FCS data at multiple distinct spots of the plasma membrane would allow direct mapping of the mobility of lipid analogues with high spatial resolution. Complementary to STED-FCS, single-molecule-tracking achieves nanometre spatial and millisecond temporal precision by following single isolated molecules in space and time over usually a large area of the membrane; however, the concomitant stochastic sampling yields low statistics and random coverage from a single measurement only. In principle, FCS-related methods such as Raster-Image-Correlation-Spectroscopy [12] , [13] , [14] and Spatiotemporal Image Correlation Spectroscopy [15] , [16] addressed this limitation by determining directed motion and diffusion coefficients from raster scanned images. However, the current image correlation methods are either limited in temporal resolution and/or require averaging over too large (>300 nm in diameter) regions of interest. A potential remedy to the limitations of image correlation spectroscopy is the rapid recording of FCS data along a line or circle, as introduced by scanning FCS [12] , [17] , [18] . Here we depict the use of scanning STED-FCS (sSTED-FCS) [19] , [20] to study spatiotemporal heterogeneity of fluorescent lipid analogues with different phase-partitioning properties in the plasma membrane of living cells. sSTED-FCS allows the distinct mapping of membrane dynamics on a several-micrometre-long scanning trajectory by a single 10-s measurement, with a maximum spatial resolution of 60 nm and submillisecond temporal resolution. We demonstrate that diffusion speeds as well as trapping characteristics of lipid analogues strongly change in space and time across the plasma membrane of living mammalian cells, independent of their preference for liquid-ordered or -disordered membrane environments, all in all contributing to an updated picture of plasma membrane organization. sSTED-FCS Similar to single-point STED-FCS, the goal of sSTED-FCS is to determine modes of diffusion (such as free versus hindered) of fluorescent reporter molecules on spatial scales smaller than the diffraction limit of light (<<250 nm). Scanning the observation spot in FCS instead of keeping it fixed can be used to, among other things, parallelize the measurement and therefore sample many spatially separated points simultaneously [12] , [17] , [18] . Applying the scanning approach to STED-FCS we intended to identify and map zones of hindered diffusion of fluorescent lipid analogues in the plasma membrane of living cells with the highest spatiotemporal resolution possible. To achieve this, we started with a confocal microscope equipped with a galvanometric beam-scanning device (Methods and Supplementary Fig. 1 ). To record fluorescence fluctuations at multiple positions quasi-simultaneously, we continuously scanned the excitation laser diffraction spot (wavelength 640 nm, spot diameter d =250 nm measured as the full-width at half-maximum (FWHM) intensity) in a circular orbit over the sample membrane at frequencies between f =1 and 6 kHz and orbital radii between r =1 and 3 μm (Fig. 1a ). With single-photon-counting detectors, this arrangement enabled the simultaneous recording of fluorescence time traces for each pixel of the scan orbit (photon counts over time for each pixel, depicted as an intensity carpet, Fig. 1b ) [17] . Circular orbits were preferred over lines because a circular scan has no back-scan and thus no de- and acceleration phases. Temporal autocorrelation of the intensity carpet then resulted in the generation of FCS data at different spatial points (FCS data at each pixel of the orbital scan, depicted as a correlation carpet, Fig. 1c ), as previously introduced in detail [13] , [17] , [18] . Independent fitting of all FCS data of the correlation carpet enabled mapping of apparent diffusion coefficients D i (calculated from the average transit times t D,i , equation (1) in Methods) for each pixel i on the orbital scan. In addition, we calculated the spatial averaged values t D =〈 t D,i 〉 i and D =〈 D i 〉 i from all pixel values (〈…〉 i denoting the averaging over all pixel values i ). To achieve subdiffraction spatial resolution, we added a 780-nm pulsed STED laser to our scanning FCS set-up featuring a central intensity zero and which confined the spatial region of the observation spot to subdiffraction size ( Fig. 1a ). Continuous tuning of the observation spot diameter from d =40 to 250 nm was possible by varying the power of the STED beam [5] , [7] . 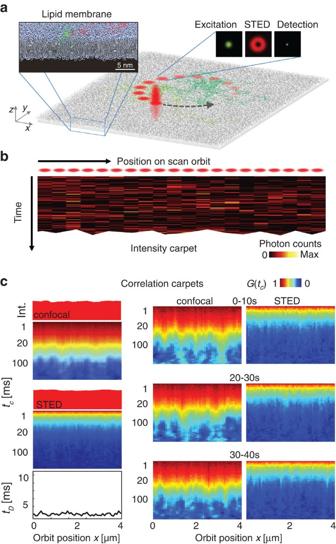Figure 1: Principle of sSTED-FCS. (a) In our experiments the spot of the excitation laser was circularly scanned over the membrane for several seconds with a radiusR>1 μm and a frequencyf=1–6 kHz, resulting in (b) a fluctuating fluorescence time trace for each pixels along the orbital path (photon counts over time for each pixel of the orbital scan, intensity carpet). The size of the observation spot was subsequently decreased to sub-250 nm diameters using increasing powersPSTEDof the STED laser, featuring an intensity distribution with a central zero (insets). (c) Correlation carpet exemplified for simulated data of free Brownian diffusion. Left panels: confocal (upper) and STED (d=80 nm, lower) data for a measurement time of 50 s. Total intensity (upper panels, normalized), correlation curves (correlation carpet, middle panels) and resulting transit timestD(lower panels, for STED only) for each pixel position of the orbital scan (scanning parameters:f=3.3 kHz, radiusR=1 μm, pixel width Δxpxl=15 nm). The correlation curvesG(tc) are presented in colour code as given in the colour scale bar. Large fluctuations in the decaying correlation curves and corresponding values oftDindicate spatial heterogeneity in diffusion environments. Right panels: correlation carpets for STED (right) and confocal (middle) at different 10-s subset of the left measurement, as labelled, possibly highlighting changes of spatial heterogeneity over time. Figure 1: Principle of sSTED-FCS. ( a ) In our experiments the spot of the excitation laser was circularly scanned over the membrane for several seconds with a radius R >1 μm and a frequency f =1–6 kHz, resulting in ( b ) a fluctuating fluorescence time trace for each pixels along the orbital path (photon counts over time for each pixel of the orbital scan, intensity carpet). The size of the observation spot was subsequently decreased to sub-250 nm diameters using increasing powers P STED of the STED laser, featuring an intensity distribution with a central zero (insets). ( c ) Correlation carpet exemplified for simulated data of free Brownian diffusion. Left panels: confocal (upper) and STED ( d =80 nm, lower) data for a measurement time of 50 s. Total intensity (upper panels, normalized), correlation curves (correlation carpet, middle panels) and resulting transit times t D (lower panels, for STED only) for each pixel position of the orbital scan (scanning parameters: f =3.3 kHz, radius R =1 μm, pixel width Δ x pxl =15 nm). The correlation curves G ( t c ) are presented in colour code as given in the colour scale bar. Large fluctuations in the decaying correlation curves and corresponding values of t D indicate spatial heterogeneity in diffusion environments. Right panels: correlation carpets for STED (right) and confocal (middle) at different 10-s subset of the left measurement, as labelled, possibly highlighting changes of spatial heterogeneity over time. Full size image First, we performed calibration measurements on supported lipid membranes to benchmark the performance of our sSTED-FCS set-up ( Supplementary Notes and Supplementary Figs 2 and 3 ). We found that the scanning frequency f has to be at least four times higher than the average transit time t D of the fluorescent molecules through the detection spot to accurately extract the diffusion dynamics by standard FCS analysis ( f >4/ t D , Supplementary Fig. 2 ). In the presented measurements, we therefore employed f =1–4 kHz. In STED-FCS experiments the observation spot sizes are decreased to observation diameters far below the diffraction limit d <250 nm, resulting in reduced values of t D (since the transit time scales with d , t D = d 2 /(8ln(2) D )). As a consequence of f >4/ t D , this puts a limit on the smallest spot size d that can be applied in sSTED-FCS. For example, in live cell experiments with fluorescent lipid analogues, which have a typical average diffusion coefficient of D =0.5 μm 2 s −1 , the smallest spot size accessible had a diameter of d =60 nm ( t D =1.3 ms, that is, a minimal frequency f =3 kHz). Similar to conventional scanning FCS we were able to determine the observation spot’s diameter d from the measurement itself using spatial correlation analysis ( Supplementary Fig. 3a ) [12] , [19] . This is an important advantage in sSTED-FCS because the observation spot size d is a function of the STED laser power P STED ( Supplementary Fig. 3b ) and previously d ( P STED ) had to be calibrated by additional measurements [5] , [7] . In addition, the obvious advantages of the scanning approach are the simultaneous observation of heterogeneity in diffusion dynamics at different points in space ( Supplementary Fig. 3c ), and the determination of average diffusion parameters ( t D or D ) with a large body of data for analysis from a single measurement only ( Supplementary Fig. 3d ). Heterogeneous diffusion of lipids in the plasma membrane Previous single-point STED-FCS experiments have exhibited distinct differences in the diffusion dynamics of Atto647N-labelled phosphoethanolamine (PE) and sphingomyelin (SM) lipid analogues (structures given in Fig. 2 ) when incorporated into the plasma membrane of living PtK2 cells. This is depicted in Fig. 3a , which shows the dependence of the apparent diffusion coefficient D ( d ) on the diameter d of the observation spot, as determined by the single-point FCS measurements for different intensities of the STED laser. The diffusion of the sphingolipid SM was hindered because of transient arrests (trapping, decrease in D towards smaller diameters d ) [5] , [6] , [7] . These arrests were most probably caused by transient interactions with immobile or slowly moving molecular entities such as proteins, with trapping times in the range of 10 ms (with on- and off-rates of 80 s −1 ) and smaller than 20-nm-sized areas in which the lipids dwelled during trapping [5] , [6] , [7] , [10] . In contrast, transient interactions of PE were much weaker (with 190 s −1 on- and large 800 s −1 off-rates), disclosing an almost free diffusion mode in the STED-FCS recordings (almost constant values of D ( d )) [5] , [6] , [7] , [10] . To further characterize the lipid-trapping sites, especially with regards to their spatiotemporal heterogeneity, we revisited these single-point STED-FCS measurements using sSTED-FCS. 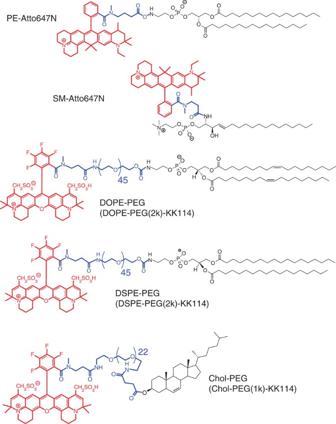Figure 2: Molecular structures of the fluorescent lipid and cholesterol analogues used in this study. Dye (red, Atto647N and KK114), linker (blue, numbers indicate numbers of repeats) and lipids/cholesterol (black). Note that the orientation and exact position of the dye with respect to the acyl chains might be different in the actual membrane environment. Figure 2: Molecular structures of the fluorescent lipid and cholesterol analogues used in this study. Dye (red, Atto647N and KK114), linker (blue, numbers indicate numbers of repeats) and lipids/cholesterol (black). Note that the orientation and exact position of the dye with respect to the acyl chains might be different in the actual membrane environment. 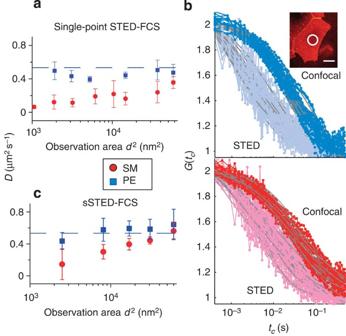Figure 3: sSTED-FCS of fluorescent PE and SM lipid analogues in the plasma membrane of live mammalian PtK2 cells. (a) Complementary single-point STED-FCS. Dependency of the apparent diffusion coefficientDon the observation area (squared diameterd2), as determined for PE (red) and SM (blue) from 35 (PE) and 52 (SM) measurements on different spots of the same and different cells (error bars=s.d. of the mean, s.d.m.). PE diffusion was mainly free (blue-dashed line exemplifies free diffusion withD=0.55 μm2s−1), while the dependence ofD(d2) of SM indicated anomalous, trapped diffusion. (b) Exemplary temporal correlation curvesG(tc) from single orbital scans over PE- (blue) and SM-labelled (red) cells for confocal (dark) and STED (sallow) recordings (d(STED)=60 nm), respectively. Each correlation curve represents one spatial position on the scanning orbit. The STED recordings reveal a larger spread (heterogeneity) for PE and SM compared with confocal resolution. In addition, the transit times of SM were on average longer for the STED data compared with PE. (Inset: scanning confocal image of a PE-labelled PtK2 cell with the white circle indicating a typical orbital scan measurement. Scale bar 2 μm). (c) The dependency ofD(d2) determined with large body of data for analysis from five sSTED-FCS within 50 s only (2,000 data points in total), revealing strongly hindered diffusion for SM and close to free diffusion for PE as ina(error bars=s.d.m.). Scanning parameters:f=3.3 kHz, radiusR=1 μm, pixel width Δxpxl=15 nm. Full size image Figure 3: sSTED-FCS of fluorescent PE and SM lipid analogues in the plasma membrane of live mammalian PtK2 cells. ( a ) Complementary single-point STED-FCS. Dependency of the apparent diffusion coefficient D on the observation area (squared diameter d 2 ), as determined for PE (red) and SM (blue) from 35 (PE) and 52 (SM) measurements on different spots of the same and different cells (error bars=s.d. of the mean, s.d.m.). PE diffusion was mainly free (blue-dashed line exemplifies free diffusion with D =0.55 μm 2 s −1 ), while the dependence of D ( d 2 ) of SM indicated anomalous, trapped diffusion. ( b ) Exemplary temporal correlation curves G ( t c ) from single orbital scans over PE- (blue) and SM-labelled (red) cells for confocal (dark) and STED (sallow) recordings ( d (STED)=60 nm), respectively. Each correlation curve represents one spatial position on the scanning orbit. The STED recordings reveal a larger spread (heterogeneity) for PE and SM compared with confocal resolution. In addition, the transit times of SM were on average longer for the STED data compared with PE. (Inset: scanning confocal image of a PE-labelled PtK2 cell with the white circle indicating a typical orbital scan measurement. Scale bar 2 μm). ( c ) The dependency of D ( d 2 ) determined with large body of data for analysis from five sSTED-FCS within 50 s only (2,000 data points in total), revealing strongly hindered diffusion for SM and close to free diffusion for PE as in a (error bars=s.d.m.). Scanning parameters: f =3.3 kHz, radius R =1 μm, pixel width Δ x pxl =15 nm. Full size image Figure 3b shows exemplary sSTED-FCS data of the diffusion of the PE and SM analogues. Lipid staining of mammalian PtK2 cells was achieved by incubating with bovine serum albumin (BSA)-complexed lipids. Measurements (that is, orbital scanning) were performed at the basal membrane of the cell, facing the cover glass, and regions with nonhomogenous fluorescence intensity (ruffles, sites of endocytosis) were avoided. Data were taken over 10 s for each of the five different STED powers ranging from P STED =0 ( d =250 nm) to P STED =110 mW ( d =60 nm) while scanning an orbit with f =3.3 kHz and radius R =1 μm. An intensity carpet was generated with Δ x pxl =15 nm pixilation resulting in >400 spatially distinct correlation curves per single data acquisition. As for the single-point measurements, sSTED-FCS showed a marked difference between PE and SM. While the confocal data of PE and SM were hardly distinguishable, the STED data of SM featured decays that were much more shifted to longer correlation lag times t c and much more stretched out than the decays for PE, which indicated a more pronounced hindrance of SM diffusion [5] , [6] , [7] . Fitting of the data resulted in >400 values of the transit time t D,i (or apparent diffusion coefficient D i = d 2 /(8(ln2) t D,i ), equation (1) in Methods) for each single measurement at the different STED powers, establishing an average and s.d. of t D = 〈t D,i 〉 i and D = 〈D i 〉 i with large body of data for analysis within only 10 s ( Fig. 3c ). This is a clear advantage over single-point STED-FCS, where a multitude of measurements, each lasting 10 s, were necessary to determine average values of diffusion parameters [5] , [6] , [7] . The dependence of D on the size of the observation spot confirmed transient molecular trapping for SM and close to free Brownian diffusion for PE as for the single-point measurements [7] . Obviously, while in earlier studies the acquisition of this dependence took hours and implied averaging over many cells and preparations, here the total recording time of the whole set of sSTED-FCS data (for five different observation sizes) was only 50 s. This allowed us to look more deeply into the characteristics of the trapping. The various sSTED-FCS data recorded for a single STED power showed a large heterogeneity in decay times ( Fig. 3b ). To explore this heterogeneity further, we investigated the spread in values of t D,i and D i in greater detail. 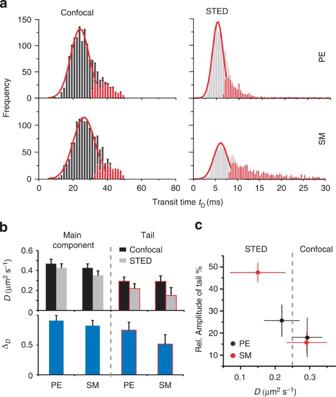Figure 4: Characterisation of lipid diffusion heterogeneities in the plasma membrane of live PtK2 cells. (a) Histograms of the transit timestDof PE (upper) and SM (lower) for confocal (d=250 nm, left) and STED (d=80 nm, right) recordings comprising 1,500 data points (different spatial positions) from six independent scans. The main peak of the histogram (black) was fitted with a single Gaussian (red line) and the residuals classified as tail (red). Note the relative increase in the tail in the SM data when resolution was increased from confocal to STED, while for PE it was unchanged. (b) Average apparent diffusion coefficientD(upper panels) of the main component and the tail (red edge) for confocal (black) and STED (grey) recordings. Lower panel depicts the ratio ΔD=DSTED/Dconfwith one indicating free diffusion and <<1 indicating hindered diffusion (error bars=s.d.m.). The ratios reveal that the tail component was caused by strong hindered diffusion because of transient molecular trapping. (c) Relative amplitude of the tail component plotted against the mean diffusion coefficient for PE (black) and SM (red). Note how the STED recordings reveal the high fraction (≈50%) of positions where SM on average diffused significantly slower than PE. Shown are the mean values (spots) and standard deviations (lines). Figure 4a plots the histogram of the values of the transit time t D,i obtained from 1,500 single-pixel data points gathered over six independent orbital scans of 30 s each. While the transit time histogram for free diffusion could be fitted by a single Gaussian distribution (as expected from Monte-Carlo simulated data, Supplementary Fig. 4 ), the histograms of PE and SM clearly contained a second slower component, whose fraction was increased when the spatial resolution was increased from the confocal d =250 nm value to, in this case, d =80 nm in the STED recordings. To characterize the slow component, we fitted the main peak of the histograms by a single Gaussian distribution ( Fig. 4a black and grey), while the data points omitted from the Gaussian fit were regarded as the tail component ( Fig. 4a red). With this classification, we estimated the average and s.d. of the apparent diffusion coefficient D for each fraction ( Fig. 4b ). While the average apparent diffusion coefficient of the main component D =0.4–0.5 μm 2 s −1 was in the range of values reported earlier from FCS measurements of supposedly nearly free Brownian lipid diffusion in the plasma membrane [7] , [21] , [22] , the average values were lower for the tail ( D =0.3 μm 2 s −1 ). When decreasing the observation spot with STED, average values of the apparent diffusion coefficient (confocal: D conf , STED: D STED ) hardly decreased for the main component of SM and PE, only slightly for the tail component of PE, but strongly for the tail component of SM. This is further quantified by the ratio Δ D = D STED / D conf , which ranges from 0.85 for the main component of PE, 0.8 for the main component of SM, over 0.75 for the tail component of PE to <0.5 for the tail component of SM. As highlighted before ( Fig. 3a,c ), values of the ratio Δ D =1 depict free, while Δ D <1 depicts increased transient trapping. [7] Consequently, the data of Fig. 4b indicate that the tail component represents membrane zones where molecules experienced strong transient trapping, while the main component represented those spatial positions where molecules were only slightly trapped or even mainly diffused freely. In total, SM seemed to be strongly trapped in 50 % of the plasma membrane area, while PE trapping occurred only at 25 % ( Fig. 4c ). Note that these conclusions could not be defined by the confocal recordings nor from six independent single-point STED-FCS measurements. Rather, for single-point STED-FCS experiments 1,500 individual acquisitions would have been required, taking several hours of measurement time and requiring several exchanges of samples. In contrast, we completed our sSTED-FCS experiments within a few minutes only on a single sample. From our previous single-point measurements we indirectly estimated that each SM lipid became trapped every 200–300 nm on average, with an average diffusion coefficient of D =0.4–0.6 μm 2 s −1 in-between the trapping events, and an average trapping probability of ∼ 55% in <80 nm large observations spots [5] , [7] . Deploying sSTED-FCS we now directly revealed the spatial pattern of the trapping sites, which was largely in agreement with the estimation from earlier single-point measurements. Figure 4: Characterisation of lipid diffusion heterogeneities in the plasma membrane of live PtK2 cells. ( a ) Histograms of the transit times t D of PE (upper) and SM (lower) for confocal ( d =250 nm, left) and STED ( d =80 nm, right) recordings comprising 1,500 data points (different spatial positions) from six independent scans. The main peak of the histogram (black) was fitted with a single Gaussian (red line) and the residuals classified as tail (red). Note the relative increase in the tail in the SM data when resolution was increased from confocal to STED, while for PE it was unchanged. ( b ) Average apparent diffusion coefficient D (upper panels) of the main component and the tail (red edge) for confocal (black) and STED (grey) recordings. Lower panel depicts the ratio Δ D = D STED / D conf with one indicating free diffusion and <<1 indicating hindered diffusion (error bars=s.d.m.). The ratios reveal that the tail component was caused by strong hindered diffusion because of transient molecular trapping. ( c ) Relative amplitude of the tail component plotted against the mean diffusion coefficient for PE (black) and SM (red). Note how the STED recordings reveal the high fraction (≈50%) of positions where SM on average diffused significantly slower than PE. Shown are the mean values (spots) and standard deviations (lines). Full size image To perceive the spatiotemporal heterogeneity of the membrane environment, we plotted the correlation data for each pixel position separately (correlation carpet, Figs 1c and 5 ). Here the decays G i ( t C ) were normalized to G i ( t C →0) and represented by a colour code, with red showing high values of G i ( t C ) at short correlation lag times t C , blue the basal offset at large t C and the decay or average transit times t D,i can be estimated from the correlation lag times of the yellowish coloured region. Vertical fluctuations of the yellowish parts over pixel position thus reveal strong fluctuations in transit times along the scanning path. For comparison, the correlation carpet is shown from two consecutive confocal and STED recordings of the same orbit. In addition, for each pixel we plotted the normalized signal intensity as well as the average transit times t D,i , as determined by averaging the signal over all times of the intensity carpet and from a fit of equation (1) (Methods) to the correlation data, respectively. A strong spatial heterogeneity in t D,i is observable. Compared with the confocal correlation carpets and the correlation carpet expected for free diffusion ( Fig. 1c ), specifically the SM sSTED-FCS data showed sites with strongly prolonged values of t D,i , which make up ∼ 50% of the space. In contrast, the correlation carpets of PE are very similar to those expected for free diffusion, indicating only weak heterogeneity and coinciding with the previous observation of almost free diffusion ( Fig. 3a ). 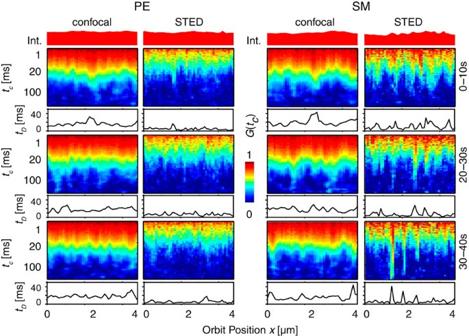Figure 5: sSTED-FCS maps the spatial and temporal heterogeneity of the fluorescent PE and SM lipid analogues in live PtK2 cells. Correlation carpets of PE (left two panels) and SM (right two panels) diffusion of confocal and STED recordings (as labelled) for consecutive 10-s measurement time intervals (as marked on the right side). Total intensity (respective upper panels, normalized), correlation carpets (respective middle panels) and fitted transit timestD(respective lower panels). The correlation carpets show the normalized temporal correlation curves corresponding to the pixel positions on the scan orbit (xaxis). The correlation amplitudeG(tc) is depicted by the colour code, while the correlation timetcis encoded in theyaxis. The respective transit times for every pixel on the scan trajectory can be estimated from the colour decay (yellow regions). Large fluctuations in transit times (tD) indicating positions of hindered diffusion are only revealed for SM in the STED recordings. The sites of hindered diffusion were smaller than 80 nm and transient, that is, they changed over consecutive time windows. Figure 5: sSTED-FCS maps the spatial and temporal heterogeneity of the fluorescent PE and SM lipid analogues in live PtK2 cells. Correlation carpets of PE (left two panels) and SM (right two panels) diffusion of confocal and STED recordings (as labelled) for consecutive 10-s measurement time intervals (as marked on the right side). Total intensity (respective upper panels, normalized), correlation carpets (respective middle panels) and fitted transit times t D (respective lower panels). The correlation carpets show the normalized temporal correlation curves corresponding to the pixel positions on the scan orbit ( x axis). The correlation amplitude G ( t c ) is depicted by the colour code, while the correlation time t c is encoded in the y axis. The respective transit times for every pixel on the scan trajectory can be estimated from the colour decay (yellow regions). Large fluctuations in transit times ( t D ) indicating positions of hindered diffusion are only revealed for SM in the STED recordings. The sites of hindered diffusion were smaller than 80 nm and transient, that is, they changed over consecutive time windows. Full size image To precisely determine the mode of diffusion (for example, values of Δ D ) on each point of the scan trajectory we would have to change the size of the observation spot during a single scan, which is at the moment not possible. However, it is very likely that the sites of slow diffusion are caused by transient molecular arrest (that is, trapping), since we can clearly correlate this observation to the results obtained from the analysis of the sSTED-FCS data of Fig. 4 , with the tail component obviously reflecting the sites of strongly hindered diffusion, and the main component the rest of space. It has to be noted that the apparent diffusion coefficients of the main component, as well as its ratio Δ D , were on average slightly lower for SM than for PE ( Fig. 4b ). Furthermore, values of t D,i of SM were on average slightly prolonged compared with PE even outside the strong trapping sites ( Fig. 5 ). Consequently, the SM lipid analogue detects sites of strong (Δ D <0.5) and weak (Δ D =0.8) transient molecular trapping alternately over space, while PE shows only weak interactions (Δ D >0.75), which were not clearly distinguishable in space. Temporal heterogeneity We next analysed the sSTED-FCS data over consecutive 10-s-time windows ( Fig. 5 ) to estimate the persistence of the trapping sites. While the basic characteristics stayed the same at each time point (that is, alternating strong and weak trapping sites), the time dependence of the data revealed strong spatiotemporal dynamics in lipid trapping. Note that the positions of the strong trapping sites as well as their total number differ between the consecutive recordings ( Supplementary Table 1 ). Their widths on the other hand hardly exceeded the 80-nm-spatial resolution of our STED recordings, that is, the average size of the strong trapping sites was below 80 nm ( Supplementary Table 1 ). Consequently, the trapping sites appeared to hardly move during the 10-s subsets (which would potentially blur the widths). Yet, the trapping sites must have persisted for up to the timescale of seconds during the 10-s subsets; otherwise, they would not have dominated the FCS decays at those points. We conclude that the trapping sites constantly appear and disappear within seconds. In addition, the trapping sites were on average separated by ∼ 200–300 nm, and also the transit times at the spatial points in between the strong trapping sites (that is, the characteristics of the presumably weak interactions) fluctuate from one 10-s subset to the next. Note that the spatial heterogeneity in total intensity of the signal (upper layers Fig. 5 ) was much less pronounced than those of the diffusion and only weakly correlated, which indicates negligible formation of dominant clusters (in detail analysed in Fig. 7 , and discussed further below). Overall, our sSTED-FCS data depict spatiotemporal variations in lipid membrane diffusion and interaction dynamics, which are inaccessible with confocal FCS recordings alone (whether single-point or scanning) and also not observable in single-point STED-FCS measurements [5] . 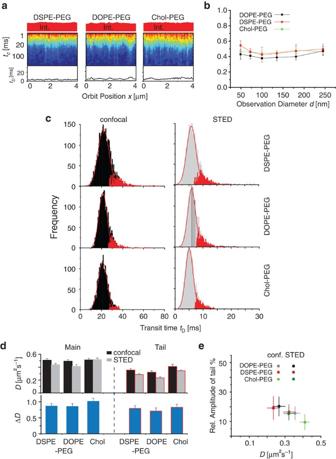Figure 6: sSTED-FCS analysis of the pegylated fluorescent lipid and cholesterol analogues in the plasma membrane of live PtK2 cells. (a) Correlation carpets of DSPE-PEG (left), DOPE-PEG (middle) and Chol-PEG (right) diffusion for STED recordings (measurement time of 10 s) as inFig. 5. Hardly any fluctuations in transit times indicate negligible sites of strong hindered diffusion. The corresponding confocal correlation carpets and time-dependent changes in correlation carpets are depicted inSupplementary Fig. 6. (b) Dependency ofDon the observation area (diameterd) for the pegylated analogues (as labelled). Shown are the average values and s.d.’s as determined by sSTED-FCS (d=250–80 nm, 1,500 data points) and single-point FCS (d=50 nm, 10 data points; error bars=s.d.m.). Despite their different phase-partitioning preference, all analogues show comparable free Brownian motion. (c) Histograms of the transit timestDof DSPE-PEG (upper), DOPE-PEG (middle) and Chol-PEG (lower) for confocal (d=250 nm, left) and STED (d=80 nm, right) recordings comprising 1,500 data points (different spatial positions) from 10 independent scans. The main peak of the histogram (black) was fitted with a single Gaussian (red line) and the residuals classified as tail (red). Note the negligible relative increase in the tail when resolution was increased from confocal to STED, indicating only weak hindrances in diffusion. (d) Average apparent diffusion coefficientD(upper panels) of the main component and the tail (red edge) for confocal (black) and STED (grey) recordings, as determined fromc. Lower panel depicts the ratio ΔD=DSTED/Dconfwith 1 indicating free diffusion and <<1 for hindered diffusion. The ratios indicate that the tail component was caused by hindered diffusion because of transient molecular trapping (error bars=s.d.m.). (e) Relative amplitude of the tail component plotted against the mean diffusion coefficient, as determined fromd. Note that the fraction of the tail component does only slightly increase from confocal to STED recordings. Shown are the mean values (spots) and s.d.’s of the mean (lines). Figure 6: sSTED-FCS analysis of the pegylated fluorescent lipid and cholesterol analogues in the plasma membrane of live PtK2 cells. ( a ) Correlation carpets of DSPE-PEG (left), DOPE-PEG (middle) and Chol-PEG (right) diffusion for STED recordings (measurement time of 10 s) as in Fig. 5 . Hardly any fluctuations in transit times indicate negligible sites of strong hindered diffusion. The corresponding confocal correlation carpets and time-dependent changes in correlation carpets are depicted in Supplementary Fig. 6 . ( b ) Dependency of D on the observation area (diameter d ) for the pegylated analogues (as labelled). Shown are the average values and s.d.’s as determined by sSTED-FCS ( d =250–80 nm, 1,500 data points) and single-point FCS ( d =50 nm, 10 data points; error bars=s.d.m.). Despite their different phase-partitioning preference, all analogues show comparable free Brownian motion. ( c ) Histograms of the transit times t D of DSPE-PEG (upper), DOPE-PEG (middle) and Chol-PEG (lower) for confocal ( d =250 nm, left) and STED ( d =80 nm, right) recordings comprising 1,500 data points (different spatial positions) from 10 independent scans. The main peak of the histogram (black) was fitted with a single Gaussian (red line) and the residuals classified as tail (red). Note the negligible relative increase in the tail when resolution was increased from confocal to STED, indicating only weak hindrances in diffusion. ( d ) Average apparent diffusion coefficient D (upper panels) of the main component and the tail (red edge) for confocal (black) and STED (grey) recordings, as determined from c . Lower panel depicts the ratio Δ D = D STED / D conf with 1 indicating free diffusion and <<1 for hindered diffusion. The ratios indicate that the tail component was caused by hindered diffusion because of transient molecular trapping (error bars=s.d.m.). ( e ) Relative amplitude of the tail component plotted against the mean diffusion coefficient, as determined from d . Note that the fraction of the tail component does only slightly increase from confocal to STED recordings. Shown are the mean values (spots) and s.d.’s of the mean (lines). 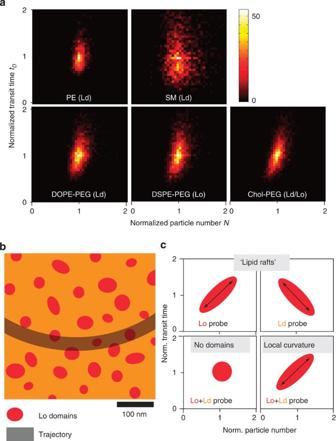Figure 7: Investigating the correlation between local mobility and concentration of lipid analogues. (a) Two-dimensional frequency histogram of pair values of transit timetDand local concentration (average particle numberNper observation spot) for the different lipid analogues (labelled, with Ld and Lo preference given) as calculated from the respective sSTED-FCS data ofFigs 4and6(1,500 data points each). For each correlation curve of the sSTED-FCS recordings values oftDandNwere determined by fittingSupplementary equation (1)to the curves. Normalized values oftD/〈tD〉 andN/〈N〉 were calculated by division with the respective average values 〈tD〉 and 〈N〉 over all pixels of each scan trajectory. Note the increased spread of values towards largetDfor SM (without a correlation, indicating trapping), and the positive correlation (tilt to the right) for the pegylated lipid analogues. (b) Scheme of potential liquid-ordered (Lo) lipid domains (red) in a Ld environment (orange) of the plasma membrane and an exemplary scanning trajectory (grey). (c) Scheme of expectedtD/〈tD〉 versusN/〈N〉 correlation plots for different scenarios. (Upper panels) In case of transient incorporation into Lo domains (‘rafts’) a positive correlation (right tilt) is expected for the Lo-probe (DSPE-PEG) and a negative correlation (left tilt) for the Ld-probe (DOPE-PEG, SM, PE), respectively. However, no Lo- and Ld-probe-specific behaviour was detected. (Lower left panel) In absence of nanodomains no correlation is expected for all probes, with an isotropic distribution for a freely diffusing probe (red). (Lower right panel) A positive correlation (right tilt) is expected for locally curved membrane regions independent of phase preference, as observed for the pegylated probes. For a detailed description of the correlation analysis and explanation of the expected distributions seeSupplementary Note 3. Full size image Figure 7: Investigating the correlation between local mobility and concentration of lipid analogues. ( a ) Two-dimensional frequency histogram of pair values of transit time t D and local concentration (average particle number N per observation spot) for the different lipid analogues (labelled, with Ld and Lo preference given) as calculated from the respective sSTED-FCS data of Figs 4 and 6 (1,500 data points each). For each correlation curve of the sSTED-FCS recordings values of t D and N were determined by fitting Supplementary equation (1) to the curves. Normalized values of t D /〈 t D 〉 and N /〈 N 〉 were calculated by division with the respective average values 〈 t D 〉 and 〈 N 〉 over all pixels of each scan trajectory. Note the increased spread of values towards large t D for SM (without a correlation, indicating trapping), and the positive correlation (tilt to the right) for the pegylated lipid analogues. ( b ) Scheme of potential liquid-ordered (Lo) lipid domains (red) in a Ld environment (orange) of the plasma membrane and an exemplary scanning trajectory (grey). ( c ) Scheme of expected t D /〈 t D 〉 versus N /〈 N 〉 correlation plots for different scenarios. (Upper panels) In case of transient incorporation into Lo domains (‘rafts’) a positive correlation (right tilt) is expected for the Lo-probe (DSPE-PEG) and a negative correlation (left tilt) for the Ld-probe (DOPE-PEG, SM, PE), respectively. However, no Lo- and Ld-probe-specific behaviour was detected. (Lower left panel) In absence of nanodomains no correlation is expected for all probes, with an isotropic distribution for a freely diffusing probe (red). (Lower right panel) A positive correlation (right tilt) is expected for locally curved membrane regions independent of phase preference, as observed for the pegylated probes. For a detailed description of the correlation analysis and explanation of the expected distributions see Supplementary Note 3 . Full size image Molecular characteristics of strong trapping sites We next investigated the molecular characteristics of the strong trapping sites, especially with regards to an increased lipid order as predicted for a ‘lipid raft’ environment. We employed a new class of fluorescent lipid and cholesterol analogues with improved properties for entering liquid-ordered and -disordered membrane regions compared with conventional fluorescent lipid analogues [23] . Saturated 1,2-distearoyl- sn -glycero-3-phosphoethanolamine (DSPE), unsaturated 1,2-dioleoyl-sn-glycero-3-phosphoethanolamine (DOPE) and cholesterol were labelled with the organic dye KK114 (ref. 24 ) at the head group via a hydrophilic PEG-linker with molecular weight 2 and 1 kDa (for structures, see Fig. 2 ). The existence of the PEG-linker dramatically improved the partitioning of the saturated phosphoglycerolipid DSPE-PEG-KK114 into liquid-ordered regions (partitioning coefficient of up to Lo% =80). As expected, the unsaturated DOPE-PEG-KK114 preferred liquid-disordered regions ( Lo% <30), while the cholesterol analogue Chol-PEG-KK114 only slightly preferred the liquid-ordered phase ( Lo% =50–60) and therefore served as a neutral reporter (for partitioning values of all analogues see Supplementary Fig. 5 ). Interestingly, none of these pegylated lipids revealed strong heterogeneity of diffusion as seen for the SM analogue in sSTED-FCS measurements ( Fig. 6a ). The complete sSTED-FCS analysis exposed even less heterogeneity (and thus less possible interactions) for these analogues than for the PE analogue without the PEG-linker ( Fig. 6b–e ). While the inert PEG-linker may hinder head-group-specific lipid interactions, the data clearly demonstrate that the trapping sites of SM were independent of preference for lipid-ordered or -disordered environments. While trapping diffusion was rather specific for the sphingolipid and slightly for the PE analogue [7] , [11] , for the noninteracting pegylated analogues, regions of slightly lowered diffusion were mainly correlated with a small increase in local concentration of these analogues ( Fig. 7a ). This indicates that the strong heterogeneities in diffusion of the SM analogue were dominated by trapping (transient binding to slow-moving or immobilized objects), while the slight variations in local diffusion of the pegylated lipids were most likely caused by local membrane curvature (pits) ( Fig. 7b ). By performing fast orbital beam scanning on a STED microscope and employing novel fluorescent lipid analogues with different phase-partitioning characteristics, we substantially expanded our previous STED-FCS experiments. In contrast to single-point STED-FCS, the beam-scanning STED-FCS (sSTED-FCS) approach reported in this paper now allows (i) recording hundreds of correlation data and calculating average values of diffusion parameters within a measurement time of a few seconds only, which previously took minutes ( Figs 3 and 4 ), (ii) studying molecular interactions at different spatial positions simultaneously and detecting neighbouring heterogeneous molecular environments with subdiffraction spatial resolution ( Fig. 5 ), (iii) studying relatively slowly diffusing molecules, which was previously biased by photobleaching ( Supplementary Fig. 7a ) and (iv) abolishing the necessity for additional calibration measurements ( Supplementary Fig. 3a ). However, compared with single-point measurements the scanning process lowers the sampling rate of an individual correlation curve, thus reducing the signal-to-noise ratio on each pixel of the correlation carpet ( Supplementary Fig. 7b ). This becomes even more pronounced for STED recordings, since with reduced observation spots the transit time and often also the signal-to-noise ratio decrease [6] . However, if the spatial information is omitted and all pixels from the whole scanning trajectory are pooled (as in Fig. 3c ), the statistical accuracy of a sSTED-FCS recording is higher than that of a nonscanned single-point FCS measurement ( Supplementary Fig. 7b ). Note that the scanning process limits the fastest diffusion processes that can be studied as well as the spatial resolution of the sSTED-FCS experiments ( Supplementary Fig. 2 ). In our case (as in usual scanning microscopes), the maximum applicable scanning frequency was several kHz (<6 kHz), that is, molecules should have a transit time through the observation spot of >0.8 ms. Lipids and fast-moving proteins on average diffuse with a coefficient D <1 μm 2 s −1 in the plasma membrane of living cells, that is, >0.8 ms transit times are only provided for observation spots of >60–80 nm in diameter. Consequently, our current sSTED-FCS measurements provided typical spatial resolutions of 60–80 nm. Sub-60-nm spatial resolution as achieved in previous single-point STED-FCS data are, however, sometimes required to more accurately characterize molecular dynamics, such as on- and off-rates of molecular complexes [6] . Therefore, single-point and scanning STED-FCS measurements may complement each other, as indicated in Fig. 7b and outlined further on. The presented sSTED-FCS experiments enabled us to shed new light on the diffusion dynamics of lipids in plasma membranes of living mammalian cells, taking fluorescent phospholipid, cholesterol and sphingolipid (SM) analogues as examples. For SM, we disclosed spatial alterations of sites of weak and strong trapping interactions ( Fig. 5 ). The strong trapping sites were transient on timescales of seconds, did not diffuse as stable entities, were separated on average by 200–300 nm and extended less than 80 nm in space ( Fig. 5 ). Taking the results of our complementary single-point STED-FCS [5] , [6] ( Fig. 3a ), we can conclude that in these strong trapping sites, SM transiently interacts with slow-moving or immobilized membrane components such as proteins, with on- and off-rates in the range of 80 s −1 . In addition, SM hardly moves during these trapping events [5] , [10] . The sSTED-FCS experiments with the new pegylated fluorescent phospholipid and cholesterol analogues revealed no significant spatial heterogeneity or trapping sites ( Fig. 6 ), independent of their preference for liquid-ordered or -disordered membrane environments ( Supplementary Fig. 5 ). This and the fact that the employed SM analogue did not prefer liquid-ordered environments in model membranes [7] , [11] let us conclude that the trapping sites observed for SM are not those molecular assemblies of high lipid order traditionally defined as ‘lipid rafts’ [1] . Rather than partitioning into ‘lipid rafts’ based on lipid-phase separation, the observed interactions of SM seem to be specific molecular complexes such as between lipids and proteins [7] . While being stable for up to seconds, these complexes render a constant exchange of SM lipid molecules in the time range of milliseconds, and with negligible movement inside. In addition to these well-separated profound assemblies, the SM lipids demonstrated the possibility of weak anomalies in diffusion at every point in space. In contrast to this trapping diffusion, pegylated fluorescent lipid and cholesterol analogues showed hardly any signs of molecular interactions. Analysis of the correlation between local mobility and concentration of the different lipid probes again indicates that with our current sSTED-FCS approach we were not able to detect phase-separated lipid nanodomains (‘rafts’; Fig. 7 ). Rather, the very weak heterogeneity of the pegylated lipid analogues was most likely caused by out-of-plane diffusion, for example, in local membrane pits ( Fig. 7b ). Despite their different partitioning preferences, all three pegylated probes showed a positive correlation between local transit times and local concentration, which contradicts the predictions based on a pattern of distinct Lo and Ld domains (compare Fig. 7 ). This persistent positive correlation could be the result of projecting locally curved membrane topography on a flat two-dimensional (2D) surface [25] , as it is carried out in the sSTED-FCS measurement. In any case, the effect of potential local membrane height differences on the diffusion of the probes is measurable but minor compared with the trapping of the SM analogue. We note that a separation into Lo and Ld phases as distinct as in ternary model membranes is not to be expected in the plasma membrane, as revealed from the significantly reduced difference in molecular order between Lo and Ld regions in phase-separated giant plasma membrane vesicles generated from living cells ( Supplementary Fig. 5 ) [11] . In addition, the resolution of our current (s)STED-FCS analysis might still be too low to observe small heterogeneity in diffusion because of more ordered nanodomains as small as <20 nm in diameter. Moreover, since our sSTED-FCS analysis so far probed only the basal plasma membrane of a limited number of cultured cell types, we may miss specialized membrane domains occurring either very sparsely or are localized on the apical or lateral side. A more complete display of the observed molecular complexes of the SM analogue could arise from expanding sSTED-FCS to the simultaneous detection of multiple colours. This would allow labelling of multiple lipids or proteins and thus could highlight the lipid interaction partners. The complete disentangling of spatiotemporal heterogeneity into different diffusion modes of, for example, actin meshwork confinement, partitioning into lipid domains and molecular trapping would require the determination of diffusion coefficients D ( d ) on multiple spatial scales d (compare Fig. 3a,c ) during a single sSTED-FCS measurement. This is not possible with the current experimental scheme, since it would require simultaneous recordings at different STED laser intensities. However, as recently demonstrated, the D ( d ) dependency can be extracted out of a single STED-FCS measurement by using pulsed excitation in conjunction with a continuous-wave STED laser and subsequently correlating fluorescence photons from increasing time delays relative to the excitation pulse (gated STED-FCS) [26] . In addition, expansion of sSTED-FCS to pair-correlation FCS [20] , [27] will highlight obstacles in the diffusion pathways of the lipids, especially along all spatial directions when combined with circular beam-scanning [13] . Beam-scanning recordings on a STED microscope can also be combined with further fluorescence fluctuation spectroscopy approaches such as fluorescence intensity distribution analysis or photon counting histograms [28] , [29] , and number and brightness analysis [30] , possibly highlighting changes in oligomerization states. The sSTED-FCS experiments shown here once again underscored the power of combining molecular fluctuation analysis with beam-scanning as well as with the tunable subdiffraction resolution of STED microscopy, thereby affording a powerful method for revealing molecular details of the cellular plasma membrane. With sSTED-FCS in hand, we should be able to expand the scope of STED-FCS experiments to study other cellular processes such as molecular transport into organelles with high spatiotemporal resolution [31] . sSTED-FCS microscope All sSTED-FCS experiments were performed on a confocal custom-built STED microscope whose main features are depicted in Supplementary Fig. 1 . The confocal unit of the STED nanoscope consisted of an excitation and detection beam path. A fibre-coupled pulsed laser diode operating at λ exc =635 nm with a pulse length of 80 ps (LDH-P-635, PicoQuant, Berlin, Germany) was used for excitation of the red fluorescence. After leaving the fibre, the excitation beam was expanded and focused into the sample using an oil immersion objective (HCXPLAPO × 100, NA=1.4, Leica Microsystems). The fluorescence emitted by the sample was collected by the same objective lens and separated from the excitation light by a custom-designed dichroic mirror (HQ640/40, AHF Analysentechnik, Tuebingen, Germany). In the following, the fluorescence was focused on a multimode fibre splitter (Fiber Optic Network Technology, Surrey, Canada). The aperture of the fibre acted as a confocal pinhole of 0.78 of the diameter of the back-projected Airy disk. In addition, the fibre 50:50 split the fluorescence signal, which was then detected by two single-photon-counting modules (APD, SPCM-AQR-13-FC, Perkin Elmer Optoelectronics, Fremont, CA). The detector signals were acquired with a single-photon-counting PC card (SPC 830, Becker&Hickl, Berlin, Germany). The confocal set-up was extended by integrating a STED laser beam. A modelocked Titanium:Sapphire laser (Ti:Sa, MaiTai, Spectra-Physics, Mountain View, USA) acted as the STED laser emitting subpicosecond pulses around λ STED =780 nm with a repetition rate of 80 MHz. The pulses of the STED laser were stretched to 250–350 ps by dispersion in a SF6 glass rod of 50 cm length and a 120-m-long polarization maintaining single-mode fibre (PMS, OZ Optics, Ontario, Canada). After the fibre, the STED beam passed through a polymeric phase plate (RPC Photonics, Rochester, NY), which introduced a linear helical phase ramp 0≤Φ≤2 π across the beam diameter. This wavefront modification gave rise to the doughnut-shaped focal intensity distribution featuring a central intensity zero. The spatial overlay between excitation and STED laser was realized with a dichroic mirror (zt740sprdc, AHF Analysentechnik). The temporal synchronization of the excitation and STED pulses was achieved by triggering the pulses of the excitation laser using the trigger signal from an internal photodiode inside the STED laser and a home-built electronic delay unit, which allowed a manual adjustment of the delay with a temporal resolution of 25 ps. The circular polarization of the STED and excitation laser light in the focal plane was maintained by a combination of λ /2 and λ /4 retardation plates in both beam paths (B. Halle, Berlin, Germany). Integration of a fast scanning unit enabled rapid scanning of the excitation and STED beam across the sample plane ( Fig. 1a ). A digital galvanometric two-mirror scanning unit (Yanus digital scan head, TILL Photonics, Gräfeling, Germany) was used for this purpose. The combination of an achromatic scan lens and a tube lens in a 4 f -configuration (focal lengths of 50 and of 240 mm, Leica, Wetzlar, Germany) realized a stationary beam position in the back aperture of the objective, preventing peripheral darkening within the focal plane at large scan ranges, such as vignetting. The maximal frequency of the Yanus scanner depended on the scan amplitude and varied between 1 and 6 kHz for scan amplitudes up to 150 μm, respectively. The hardware and data acquisition were controlled by the software ImSpector ( http://www.imspector.de/ ). Data acquisition, processing and analysis In order to calculate the correlation function from the detected signal at each position of the scanned orbit, it was crucial to accurately determine the spatial origin of each detected photon. The data acquisition was controlled by the software ImSpector, which initialized and generated the voltage waveforms for the scan movement and synchronized the data acquisition by the single-photon-counting PC card. Figure 1 depicts a typical recording in a scanning FCS experiment. Here the laser spots were continuously scanned along a circular trajectory of radius R =1.2 μm and frequency f =4 kHz ( Fig. 1a ). The scan trajectory was subdivided into a defined number of pixels N pxl (50–400), and the intensity fluctuations in time for each pixel were stored as a 2D array (intensity carpet, I ( i , t ) for each pixel i , Fig. 1b ) [12] . Since the diffusion of the particles does not depend on the incident laser light (which we can safely assume, following previous control measurements, even for the strong STED laser light [5] , [6] , [7] ), we evaluated the temporal fluctuations for each column of the intensity carpet by FCS. Using a multiple-tau algorithm, we correlated each column of the recorded intensity I ( i , t ) yielding a temporal correlation curve G i ( t c )=〈 I ( i , t ) I ( i , t + t c )〉/〈 I ( i , t )〉 [2] for each pixel i (correlation carpet, Fig. 1c , with t c denoting the temporal correlation time lag and 〈…〉 averaging over time t ) [12] , [13] . Since the laser spots were scanned continuously along the scan trajectory, we had to choose pixel sizes Δ x pxl much smaller than the diameter d of the observation area (as outlined in the Supplementary Notes , Methods). Only in this case, the observation spot was still sufficiently well approximated by a Gaussian detection profile and the theoretical model of a single-spot FCS measurement could well be applied: where N i is the particle number (that is, the mean number of fluorescent molecules in the detection spot, which is proportional to the concentration divided by the measurement volume (or area for 2D samples)) and t D,i is the average transit time of the fluorescent molecules diffusing through the observation area. Fitting the above equation to the FCS data resulted in a value of the average transit time t D,i or the apparent diffusion coefficient D i = ω 0 2 /(4 t d,i )= d 2 /(8 ln(2) t d,i ), and the particle number N i for each pixel i of the circular scan. Here ω 0 is the 1/ e 2 radius and d = ω 0 √(1 × ln(2)) the diameter (given as the FWHM) of the observation spot for a given STED intensity, which is either determined from measurements of the free-diffusing lipid analogue in a supported lipid bilayer (Methods) or from the spatial correlation analysis (equation (3)). One sSTED-FCS measurement thus resulted in N pxl values of t D,i or D i , which, on one hand, allowed the investigation of diffusion characteristics over space (by plotting t D,i or D i along the different spatial coordinates i of the circular scan) and, on the other hand, allowed the determination of average values t D =〈 t D,i 〉 i and D =〈 D i 〉 i (with 〈…〉 i denoting the averaging over all N pxl pixel values i ) and s.d.’s with large body of data for analysis. Note that we in our sSTED-FCS analysis discarded the introduction of a parameter for anomalous diffusion, since we were mainly interested in values of the average transit time t D,i , which is accurately well extracted using equation (1) [22] . The introduction of an additional anomaly parameter hardly changed the results obtained for t D,i , but rather decreased the accuracy of its determination, a reason why we kept the number of free fitting parameters to a minimum. In previous single-point STED-FCS experiments, we had introduced an anomaly parameter to extract anomalies in diffusion from a single FCS curve [5] . An anomaly in diffusion is however already well extracted from a single sSTED-FCS analysis, since hundreds ( N pxl ) of FCS curves are simultaneously gathered. Hence, we used the heterogeneity in the distribution of the resulting values of t D,i (or D i ) as a measure for the respective extent of anomalous diffusion (compare Fig. 4 ). All data analysis procedures were implemented into Matlab (The MathWorks Inc). Spatiotemporal correlation analysis The spatiotemporal correlation data of our sSTED-FCS experiments ( Supplementary Figs 2 and 3 ) were calculated by the 2D spatiotemporal correlation function G ( x , t c )=〈 I ( i , t ) I ( i + x , t + t c )〉/〈 I ( i , t )〉 i,t 2 of the intensity carpet I ( i , t ) with x and t c denoting the spatial and temporal correlation lag times, respectively, and 〈…〉 i,t indicating the averaging overall spatial i and temporal t recordings. An important prerequisite for this analysis is that the spatial and temporal separations between adjacent pixels and subsequent scans is constant within the intensity carpet. As for the temporal correlation, for pixel sizes Δ x pxl much smaller than the diameter d of the Gaussian-shaped observation spot profile, the theoretical model of the spatiotemporal correlation function can be calculated according to [12] . Here D is the apparent diffusion coefficient, d the diameter of the observation spot (given as the FWHM as before) and v the scan velocity. The spatiotemporal correlation function is effectively split into two terms. The first term expresses the correlation because of the diffusional movement of the particles, rendering the average transit time t D = d 2 /(8 ln(2) D ), as it is extracted from conventional FCS measurement (equation (1)). The second exponential term in contrast reflects the correlation because of the scanning movement of the observation area. For a scan velocity v that is much faster than the diffusion ( v >> D / d , which is a prerequisite of any scanning FCS measurement [12] , [17] , [18] ), this expression decouples D from d , and the spatial correlation at zero lag time t c =0, G ( x ,0), can be written as realizing a straightforward determination of d . Hence, with the scan velocity v known from the scanning speed, fitting both equations (2) and (3) to the experimental data allowed us to simultaneously determine the two quantities D and d in a single measurement, making the characterization of d from control experiments on model membranes obsolete [19] . Sample preparation 1,2-dioleoyl-sn-glycero-3-phosphocholine (DOPC) and Ganglioside GM1 (Ovine Brain) were purchased from Avanti (Avanti Polar Lipids Inc., Alabaster, Alabama, USA). Cholera Toxin B (CtxB) subunit was purchased from Sigma-Aldrich and labelled with the amine reactive dye KK114-NHS [24] (now AbberiorSTAR, Abberior) according to the standard protocol, resulting in less than or equal to two dyes per CtxB. The two lipid analogues labelled with the organic dye Atto647N, N-(Atto647N)-1,2-dipalmitoyl-sn-glycero-3-PE (head-group labelling; DPPE-Atto647N or simply PE) and N-(Atto647N)-sphingosylphosphocholine (acyl-chain replacement; SM-Atto647N or simply SM) were purchased from Atto-Tec (ATTO-TEC GmbH, Siegen, Germany). The lipids labelled with the organic dye KK114, PE-KK114, DSPE-PEG(2k)-KK114 (or simply DSPE-PEG, head-group labelling), DOPE-PEG(2k)-KK114 (or simply DOPE-PEG, head-group labelling) and Cholesterol-PEG(1k)-KK114 (or simply Chol-PEG) were synthesized as described previously [23] using starting compounds DSPE-PEG(2000)-NH2, DOPE-PEG(2000)-NH2 (Avanti Polar Lipids), Cholesterol-PEG(1000)-NH2 (Nanocs Inc., NY, USA) and the amine reactive dye KK114-NHS [24] . The molecular structures of all fluorescent lipid analogues are depicted in Fig. 2 . Supported lipid bilayers were prepared as described in ref. 23 . Glass Cover slides were cleaned in a 3:1 mixture of concentrated H 2 SO 4 and 30% H 2 O 2 . After acid cleaning, the glass slides were extensively rinsed with pure water and then stored in water for not longer than a week. Finally, the single phase liquid-disordered bilayers were made by spin-coating (2,000 r.p.m.) 20 μl of DOPC (2 g l −1 in methanol–chloroform). After 10 min solvent evaporation under vacuum the sample was hydrated with 150 mM NaCl, 10 mM TRIS/HCl pH 7.4 and rinsed several times until a clean single bilayer remained on the surface. For the sSTED-FCS experiments of Supplementary Fig. 2 , 0.01% of PE-KK114 was added to DOPC, and for those of Supplementary Fig. 3 0.1% of GM1 were added to DOPC, 100 nM of the labelled CtxB added after spin-coating and unbound CtxB rinsed off after 5 min of incubation. The mammalian PtK2 cell line (epithelia kidney cells from Potorous tridactylis ) was the same as in previous measurements [5] , [6] , [7] , [10] , [11] and was cultured in Dulbecco’s Modied Eagle Medium (DMEM) supplemented with 5% fetal calf serum, 100 U ml −1 penicillin, 100 μg ml −1 streptomycin (all Invitrogen) and 1 mM pyruvate (Sigma) at 37 °C kept within a water-saturated atmosphere of 5% CO 2 in air. Before the experiments, cells were seeded on standard glass coverslips (no. 1.5, that is 10–18 mm in thickness) to a confluence of ∼ 70% and grown at 37 °C for 24 h. Incorporation of the fluorescently labelled lipid analogues to the plasma membrane of live PtK2 cell was performed as described in ref. 5 . The passive incorporation of the lipids was facilitated via the formation of a bovine serum albumin (BSA) complex of the lipid analogue. The BSA complex was prepared by drying 100 nmol of the lipid stock solution under a stream of nitrogen. The dried lipids were then dissolved in 5 μl of ethanol and subsequently diluted in 1 ml of defatted BSA solution (7 g l −1 defatted BSA in DMEM without phenol-red buffered with 10 mM HEPES, pH 7.4). The stock solution of the pegylated cholesterol analogue was prepared in PBS without BSA. The BSA–lipid–stock solution was then diluted in HDMEM to a final concentration of 5–500 nM, varying for the individual fluorescent lipid analogues. Previous to the fluorescent labelling, the cells were washed in warm HDMEM and incubated with the diluted BSA–lipid solution for 5 min at 37 °C. Afterwards, cells were washed in HDMEM and mounted into a microscope chamber. Measurements were taken at room temperature and completed after 30 min before any significant morphological changes in the cell occurred. All measurements were carried out for at least 10 s, providing a correlation time longer than two orders of magnitude times the typical transient time of the labelled lipids through the confocal observation area. As detailed previously [5] , [7] , [9] , we ensured a non-detectable (at least by STED-FCS) influence by the dye label (apart from an altered liquid-ordered partitioning preference), and that the observation times were given by the transit times through the observation spot and not shortened because of photobleaching, and that biasing effects by the excitation or STED light because of photobleaching, heating or other (nonlinear) effects and diffusion of nonintegrated lipids (or dye tags) could be excluded. sSTED-FCS simulations To estimate the significance of the spatiotemporal heterogeneities observed in our sSTED-FCS experiments, we performed computer simulations of free Brownian diffusion. Simulations of sSTED-FCS were run in MATLAB. Free diffusion of single particles in an 8 × 8-μm simulation box with periodic boundaries was simulated by adding random step sizes for the x and y coordinates independently drawn from a normal distribution with σ =√(2 D × Δ t ), where D is the lateral diffusion coefficient and Δ t the sampling time. Fluorescence fluctuations of each pixel on a circular trajectory centred in the middle of the simulation box were calculated as described in ref. 32 . The average counts per molecule, which is a function of the properties of the fluorescence dye and the collection efficiency of set-up, and the dark count rate (noise) were adjusted to match the experimental conditions. Partitioning experiments Partitioning preference of the fluorescent lipid analogues into less and more ordered membrane regions (liquid-disordered Ld and liquid-ordered Lo membrane phases) was determined from fluorescence scanning experiments (Zeiss 710 confocal) on phase-separated giant unilamellar vesicles of a ternary lipid mixture (DOPC:SM:cholesterol (2:2:1)) and on phase-separated giant plasma membrane vesicles, generated from PtK2 cells [33] . The Lo-partitioning coefficient Lo% = F (Lo)/[ F (Lo)+ F (Ld)] was calculated from the fluorescence intensity profile of a line scan through Lo and Ld phases where the Ld phase was marked by the fluorescent membrane molecule Fast-DIO (Invitrogen) [11] . How to cite this article : Honigmann, A. et al. Scanning STED-FCS reveals spatiotemporal heterogeneity of lipid interaction in the plasma membrane of living cells. Nat. Commun. 5:5412 doi: 10.1038/ncomms6412 (2014).